Caribbean-wide decline in carbonate production threatens coral reef growth Global-scale deteriorations in coral reef health have caused major shifts in species composition. One projected consequence is a lowering of reef carbonate production rates, potentially impairing reef growth, compromising ecosystem functionality and ultimately leading to net reef erosion. Here, using measures of gross and net carbonate production and erosion from 19 Caribbean reefs, we show that contemporary carbonate production rates are now substantially below historical (mid- to late-Holocene) values. On average, current production rates are reduced by at least 50%, and 37% of surveyed sites were net erosional. Calculated accretion rates (mm year −1 ) for shallow fore-reef habitats are also close to an order of magnitude lower than Holocene averages. A live coral cover threshold of ~10% appears critical to maintaining positive production states. Below this ecological threshold carbonate budgets typically become net negative and threaten reef accretion. Collectively, these data suggest that recent ecological declines are now suppressing Caribbean reef growth potential. Coral reefs form some of the planet’s most biologically diverse ecosystems, providing numerous ecosystem goods and services [1] . Much of this functionality is linked to the structure of the reefs themselves, that provide both complex 3-dimensional habitats, and breakwater structures that modify wave energy regimes and act as protective breakwaters for adjacent shorelines. However, at the global scale, coral reefs have been severely impacted over recent decades by multiple human disturbances [2] . Coral cover is estimated to be declining by 1–2% per annum across the Indo-Pacific [3] , and has already declined by an average of ~80% in the Caribbean since the mid-1970s ( [4] ). Commensurate with these declines has been a loss of reef architectural complexity [5] . Climate change is an additional threat. Elevated sea-surface temperatures have caused widespread coral bleaching [6] , and increasing atmospheric CO 2 concentrations are projected to drive further warming and ocean acidification [7] . These changes have important implications for coral reef ecosystems generally, but it has also been suggested that such changes will result in lower rates of reef carbonate production [8] , which will limit the potential for coral reef growth in the future and, potentially, lead to a collapse of reef structures [7] . Quantitative data to support these ideas are essentially absent, but clearly any such loss of vertical growth capacity will profoundly inhibit the ability of reefs to keep pace with projected increases in sea-level, and severely impede many of the ecosystem functions and services that are underpinned by reef structures and their associated topographic complexity. The geomorphic state of reefs, as measured by the development and maintenance of their topographically complex carbonate structures, is dependent upon the net accumulation of calcium carbonate. This is a function of the balance between constructional (for example, coral and coralline algal production) and erosional (biological and physical erosion) processes [8] . Where the balance is positive, net accumulation (and thus reef growth) is typical, but where the system switches to a net negative state, such as may happen under conditions of high biological erosion, net erosion of reef structures can occur [8] . Short-term transitions of this type have been documented at individual sites following local disturbances [9] . Key questions that arise, however, are: what impacts have regional scale changes in coral reef ecology had on the carbonate production states of shallow-water reef habitats? how do carbonate production rates calculated for contemporary ecosystems compare with those established over mid- to late Holocene timescales, that is, how do they compare with rates calculated for the period pre- major human pressure in the region? and what implications do these changes have for reef growth potential in the future? Here, we report contemporary rates of reef carbonate production and bioerosion measured from 101 transects on 19 coral reefs in 4 countries (Bahamas, Belize, Bonaire and Grand Cayman) from across the Caribbean ( Fig. 1 ). We then use these data to determine net rates of biologically-driven carbonate production (kg CaCO 3 m −2 year −1 ) and resultant accretion rates (mm year −1 ) ( Methods ). Within these countries data were collected from a range of common Caribbean reef habitats: nearshore hardgrounds, Acropora palmata habitats, Montastraea spur-and-groove zones, fore-reef slopes, and deeper (18–20 m) shelf-edge Montastraea reefs. The countries examined occur in different regions with respect to prevailing wave energy/hurricane frequency [10] , and thus some degree of inherent variability in their background ecological conditions, as a function of recent disturbance history, must be assumed. However, the general ecological condition of most of the sites examined was remarkably consistent, and typified the spectrum of reef ecological states presently observed in shallow-water habitats across much of the region [4] , [11] : on most of the reefs live coral cover was less than ~25–30% (often markedly so); most shallow water sites (<10 m) were devoid of, or had very low cover of, living branched Acropora species (historically a key reef building taxa in the region and one capable of high carbonate production rates) [12] ; macroalgal cover was high (often exceeding 40%); and abundances of key substrate grazing taxa (urchins and parrotfish) were low. The notable exceptions were a few sites in Bonaire, where live coral cover was higher (in places around 40%), and this is consistent with reports that consider Bonaire as being relatively ‘healthy’ compared with other Caribbean reefs, and its designation as having the ‘most pristine’ reefs in the Caribbean [13] . At each of the sites examined we used the ReefBudget census-based methodology [14] , to measure biologically-driven carbonate production and erosion, and thus to determine net production rates ( G , where G =kg CaCO 3 m −2 year −1 ) [15] . 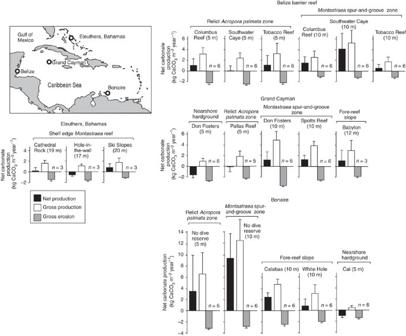Figure 1: Caribbean study sites and reef carbonate production rates. Location of study sites across the Caribbean and plots showing gross carbonate production and erosion, and net production rates (kg CaCO3m−2year−1) for each study reef. Data are grouped by country.n=number of transects per reef site. Figure 1: Caribbean study sites and reef carbonate production rates. Location of study sites across the Caribbean and plots showing gross carbonate production and erosion, and net production rates (kg CaCO 3 m −2 year −1 ) for each study reef. Data are grouped by country. n =number of transects per reef site. Full size image Net reef carbonate production across the Caribbean Net carbonate production rates across our study reefs ranged from −1.77 to 9.51 G. At the reef scale 21% of reefs had net negative budgets (range: −1.77 to −0.14 G) and 26% had positive budgets but were still below 1 G. Only 5% of reefs had net rates >5 G ( Fig. 1 ; see Supplementary Table S1 ). The most productive reefs were inside the ‘no dive reserve’ in Bonaire, where average net production was +3.63 G (5 m depth) and +9.53 G at 10 m depth ( Fig. 1 ). At the transect scale 37 of the 101 transects had negative budgets and 22 had rates between 0–1 G. Only nine transects had rates >5 G and just 5 rates >10 G. The remainder were between 1 and 5 G ( Fig. 2a ). Net carbonate production rates vary between and within habitats. Montastraea spur-and-groove habitats had the highest G values (mean 3.0 G; range −0.47 to 16.68 G; Fig. 2b ): all other habitats had mean G values <1.5 (for individual ranges see Fig. 2b ). However, pooling of data by country and habitat ( Fig. 2c ) indicates significant intra-regional variability. Net production rates in Montastraea spur-and-groove habitats in Bonaire range from 3.51 to 16.68 G and are significantly higher ( F =11.485, P <0.001) than in Belize (range: −0.46 to 10.68 G) and Grand Cayman (range: −0.47 to 4.15 G), a finding consistent with reports that cite Bonaire as having among the best remaining reefs in the Caribbean [13] , although recent reports suggest even these reefs are on a declining trajectory [16] . Net production rates in shallow A. palmata habitats are, on average, also higher in Bonaire (range: −1.74 to 15.25 G) compared with those from Belize (range: −1.33 to 3.68 G) and Grand Cayman (range: −1.54 to 1.53 G), but are not significantly different. 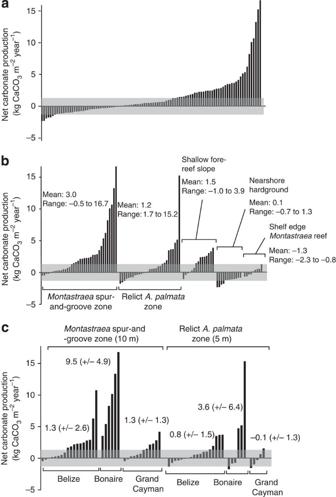Figure 2: Trends in net reef carbonate production rates at the transect level across the Caribbean. Plots showing trends in net carbonate production rates (kg CaCO3m−2year−1) measured at the transect level. (a) All data, all sites; (b) data pooled by habitat type; (c) data for the two main shallow water habitats pooled at the country level. Grey bands denote the critical transition zone (where budgets fall within the range ±1 kg CaCO3m−2year−1) and within which reef accretion is likely to either stall or move into net erosional states. Figure 2: Trends in net reef carbonate production rates at the transect level across the Caribbean. Plots showing trends in net carbonate production rates (kg CaCO 3 m −2 year −1 ) measured at the transect level. ( a ) All data, all sites; ( b ) data pooled by habitat type; ( c ) data for the two main shallow water habitats pooled at the country level. Grey bands denote the critical transition zone (where budgets fall within the range ±1 kg CaCO 3 m −2 year −1 ) and within which reef accretion is likely to either stall or move into net erosional states. Full size image Relationships between reef ecology and net production Linear mixed effects (LME) models (see Methods ) indicate that live coral cover significantly affected G ( F =159.1, P <0.001) across all reef habitats and water depths ( Fig. 3a ) and that the relationship was not significantly different between the major shallow water reef habitats examined ( Fig. 3b ). Most importantly, however, these data sets collectively indicate that Caribbean reefs typically shift into negative net production states ( G <0) when live coral cover falls below ~10%. In our approach this threshold level is calculated as a function of the true three-dimensional area of the reef and is not simply derived from planimetric representations of the reef surface [17] . A live coral cover threshold of around 10% can thus be regarded as an important boundary point for maintaining positive G values. The precise point at which an individual reef will move into a net negative production state will inevitably vary, in part as a function of the types of coral taxa present (which have variable calcification rates), but also depending upon the numbers and types of bioeroding taxa (urchins, parrotfish and so on) present, whose potential to erode the substrate also varies. For this reason it is most sensible to regard the 10% figure as a boundary point, rather than a fixed metric, around which reefs are likely to be budget neutral (see hatched zone in Fig. 3 ). We note, however, the high number of reefs in our study where live coral cover is close to this level, suggesting that many Caribbean reefs may presently be in, or are very close to being in, budget neutral states (that is, states of ‘accretionary stasis’) [8] . Thus, although the basic facets of reef geomorphic integrity presently remain intact on many Caribbean reefs, the continued maintenance of topographically complex reef structures into the future may be more questionable. 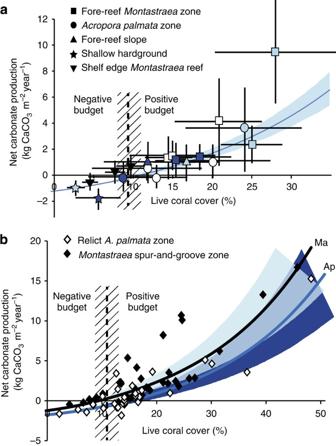Figure 3: Relationships between live coral cover and carbonate production rates across the Caribbean. Plots showing the relationships between live coral cover and carbonate production rates (kg CaCO3m−2year−1) at sites across the Caribbean. (a) Average net carbonate production against live coral cover for all 19 reefs delineated by habitat type. Black symbols—Bahamas, white symbols—Belize, light blue symbols—Bonaire, dark blue symbols—Grand Cayman. Vertical and horizontal bars are s.d. of data for each site. Best fit regression line and 95% confidence intervals shown in pale blue. (b) Net carbonate production against live coral cover at the transect level within the two major shallow water Caribbean reef habitats. Best fit regression line and 95% confidence intervals shown in dark blue forA. palmatareefs, and in pale blue forMontastraeaspur-and-groove reefs. Vertical hatched bands denote the critical transition zone, around 10% live coral cover, below which reefs typically start to move into net erosion states. Figure 3: Relationships between live coral cover and carbonate production rates across the Caribbean. Plots showing the relationships between live coral cover and carbonate production rates (kg CaCO 3 m −2 year −1 ) at sites across the Caribbean. ( a ) Average net carbonate production against live coral cover for all 19 reefs delineated by habitat type. Black symbols—Bahamas, white symbols—Belize, light blue symbols—Bonaire, dark blue symbols—Grand Cayman. Vertical and horizontal bars are s.d. of data for each site. Best fit regression line and 95% confidence intervals shown in pale blue. ( b ) Net carbonate production against live coral cover at the transect level within the two major shallow water Caribbean reef habitats. Best fit regression line and 95% confidence intervals shown in dark blue for A. palmata reefs, and in pale blue for Montastraea spur-and-groove reefs. Vertical hatched bands denote the critical transition zone, around 10% live coral cover, below which reefs typically start to move into net erosion states. Full size image Our estimates of carbonate production rates measured on reefs from across the Caribbean suggest that observed regional scale changes in benthic ecology (especially coral cover loss) have resulted in low net rates of carbonate production. These metrics are consistent with projected budgetary impacts of reef ecological decline [8] . However, quantitative data to support such assertions have, until now, been limited, and clear linkages between the ecological state of reefs and their past and present growth potential have remained unresolved. Key questions thus arise about how these measured contemporary rates compare with those measured over historical and geological timescales in the region. Insights into recent changes in the geomorphic performance of reefs can be gained through comparison of our contemporary data with measures of reef production through the mid- to late Holocene using both early budget data sets from the 1960s and 70’s, but also long-term (centennial to millennial timescale) reef core data sets. Gross carbonate production estimates from shallow water (0–10 m depth) Caribbean fore-reef habitats, before recent changes in reef ecology, are reported to have been in the range 10–17 G [12] , although rates of ~10 G are considered a low end rate for shallow water habitats with high branched coral cover [12] . Our data are markedly below this minimum rate, averaging ~3.5 G across all sites/depths, but ~40% of sites have gross production rates of <2 G. Adopting the conservative (low end) 10 G production value as a benchmark, the average production rates we have calculated are >50% lower than rates calculated for mid- and late-Holocene periods and in many cases are markedly lower (especially in the habitats previously dominated by A. palmata ). High gross production rates close to high historical values (>10 G) were calculated only for the few sites with high live coral cover dominated by healthy Montastraea populations. In contrast to earlier states of Caribbean reef ecology, where high carbonate production rates were driven by corals of the genera Acropora and Montastraea , there is thus now an essentially monospecies dependency on corals of Montastraea complex to maintain positive production states at the sites where rates remain high. These remaining high productivity sites may thus quickly transition to very low net production states if regional declines in Montastraea populations continue [18] . With regard to net carbonate production rates our data indicate that while ~65% of transects surveyed exhibited positive net carbonate production states, 58% had rates <1 G and 37% were net negative. Net production rates exceeding 5 G were calculated for only 9% of transects. The average across all transects is 1.5 G. When compared with the most detailed Caribbean budget undertaken at Bellairs reef (Barbados), where a net rate of 4.5 G was measured [19] , [20] , our rates are very low (especially given that the Bellairs reef had already lost most of its high productivity A. palmata cover). However, our measured net production values are in accord with those from other reefs affected by major ecological decline (for example, St Croix: 0.9 G (ref. 21 ) and N. Jamaica: 1.2–1.8 G (ref. 22 ). It is pertinent to note here that we may actually underestimate gross erosion rates because endolithic bioerosion is difficult to quantify [14] , with the consequence that actual net production values for many of our sites may be even lower than we calculate. It is also of significant interest to examine what our contemporary production rates mean in terms of reef accretion potential and to compare these with long-term rates as measured in Holocene reef core records from the Caribbean. To do this we compared our data with published accretion rates derived from a range of depth-stratified intervals in cores (<5, 5–10, >10 m palaeodepths) [23] and which thus equate to the range of depth intervals we examined across the Caribbean. We converted our production rate estimates to potential accretion rates (mm year −1 ) using established approaches based on carbonate density and the average porosity of reef framework [23] , [24] , but also accounted for the re-incorporation of a proportion of bioerosion-derived sediment into the framework ( Methods ). The resultant average accretion rate across our sites is 1.36 mm year −1 but is highly variable (range: −1.17 to 11.93 mm year −1 ). The very high end rates at our ‘healthiest’ sites were thus comparable with those calculated for some Holocene high productivity Acropora dominated reefs in the Caribbean, for example, Alacran reef, Mexico: 12 mm year −1 (ref. 25 ). However, for transects <5 m depth, average Holocene accretion rates across the Caribbean were nearly an order of magnitude higher than those measured in our study (3.6 mm year −1 compared with 0.6 mm year −1 ), and at depths of 5–10 m our rates were nearly 50% lower than the Holocene average (2.1 compared with 3.8 mm year −1 ; Fig. 4 ). At the individual habitat level, our data sets indicate average contemporary accretion rates within A. palmata habitats of 1.2 mm year −1 , and in the Montastraea spur-and-groove habitats of 2.3 mm year −1 . These compare with long-term equivalent Holocene averages of 3.8 and 3.1 mm year −1 , respectively [23] . We therefore calculate that accretion rates in contemporary A. palmata habitats are ~65–70% lower than the Holocene average, and ~25% lower in Montrastraea habitats. Furthermore, our current estimates of accretion are at the optimistic end of the spectrum because they do not factor for any post-production export of carbonate [26] . 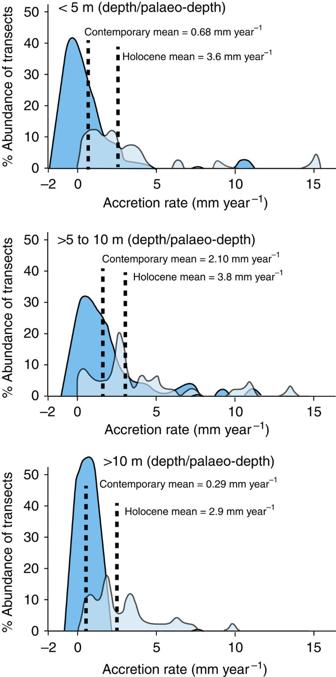Figure 4: Comparison of contemporary and Holocene reef accretion rates across the Caribbean. Plots showing a comparison of depth-related patterns of contemporary and Holocene reef accretion (mm year−1) across the Caribbean. Contemporary accretion rates from sites in this study (dark blue plots) compared with those calculated for individual depositional horizons in Holocene reef cores (light blue plots) from sites across the Caribbean/Western Atlantic (data in ref.23). Data are plotted as % abundance of core intervals/sites against measured accretion rate. Net negative rates are calculated for many of the modern sites implying conditions of net reef erosion. Figure 4: Comparison of contemporary and Holocene reef accretion rates across the Caribbean. Plots showing a comparison of depth-related patterns of contemporary and Holocene reef accretion (mm year −1 ) across the Caribbean. Contemporary accretion rates from sites in this study (dark blue plots) compared with those calculated for individual depositional horizons in Holocene reef cores (light blue plots) from sites across the Caribbean/Western Atlantic (data in ref. 23 ). Data are plotted as % abundance of core intervals/sites against measured accretion rate. Net negative rates are calculated for many of the modern sites implying conditions of net reef erosion. Full size image Our results provide strong evidence that recent declines in live coral cover, and associated changes in benthic community composition on Caribbean coral reefs, are now compromising reef growth. Net carbonate production and accretion rates in shallow water Caribbean reef habitats are below long-term rates determined from Holocene core-derived values, and below rates calculated for Caribbean reefs before the recent ecological declines caused (largely) by disease and bleaching-induced coral. That is, they are below rates determined in pre-1970s data sets. Although there is clear evidence that reef growth rates through the Holocene have been variable [23] , and that some reefs effectively ceased accreting before the era of recent human-induced decline [27] , [28] , our data suggest that ecological declines on coral reefs across the Caribbean are severely impeding carbonate production and reef accretion potential in these critical shallow water habitats. This recent shift has important implications for the maintenance of reef framework and for the ability of reefs to respond positively to future sea-level rise. A further implication here is that although reef accretion rates are generally assumed to be higher in ‘shallow’ (<10 m) compared with ‘deep’ (>10 m) reef environments, the relative difference between the two may be changing as shallow water habitats experience relatively greater rates of ecological decline. Many shallow water reefs across the Caribbean are therefore probably at an accretionary threshold. Although there is no solid evidence for significant regional scale loss (erosion) of the underlying framework structure of reefs at present, the geomorphological complexity of many reef surfaces is clearly declining [5] , and our data suggest that under present trends this may ultimately extend to loss of the underlying (Holocene) structure. The potential for production states to revert to those typical of the past is likely to be highly site specific, but also strongly influenced by external factors. For example, if communities of branched Acropora recover, as observed at a few select sites in the region [29] , then relatively rapid shifts back to higher net production states may occur. However, where communities persist in altered coral community states, dominated by ‘weedy’ taxa such as Porites astreoides and Agaricia agaricites [3] , [30] , then more persistent low net (or negative) erosional regimes will likely endure. Differential exposure to high magnitude physical disturbance events across the region, which may increase as oceans warm [31] (but see also ref. 32 ), and uncertain responses to projected more frequent bleaching episodes, will also inhibit positive budget transitions. That many of the reefs that retain high carbonate production rates (>5 G) have an essentially monospecific dependency on corals of the Montastraea complex is an additional pressing concern. Loss of these corals would have major consequences for reef growth potential in the future. Finally, given that coral cover is also on a general downward trajectory on reefs throughout the Indo-Pacific region [3] , our findings raise important questions about contemporary reef growth potential globally, and about how resilient the geomorphic structure of reefs will be if coral cover continues to decline in the face of changing environmental and climatic regimes. Quantifying gross and net carbonate production and erosion rates We collected data on gross carbonate production and erosion rates to determine net carbonate production (G, where G =kg CaCO 3 m −2 year −1 ) [15] and accretion rates (mm year −1 ) from four countries across the Caribbean (Bahamas, Belize, Bonaire and Grand Cayman) between November 2010 and March 2012. As we were interested in determining the relative importance of different biological carbonate producers and eroders in different environments, and examining these in the context of ecological change, we adopted the ReefBudget census-based methodology to determine rates of G [14] . To derive measures of benthic carbonate production we used census approaches to determine abundance of benthic carbonate producers and calculated carbonate production rates using published linear extension and density metrics for individual species (or nearest equivalent species), following ref. 14 . Estimates of substrate erosion rates were based on a census of bioeroding sponge tissue cover, available substrate for microendolithic bioerosion, metrics on species and size class of bioeroding urchins, and metrics on species-size-life phases of bioeroding parrotfish locally calibrated with bite rate data. Comparing net production rates within and between reef sites A one-way ANOVA, with Bonferroni multiple pairwise comparisons, was used to test for differences in G between countries. However, the spatial nature of the data meant that transects within reefs were likely to be more similar to each other than to transects on other reefs. The data were also unbalanced as the number of transects surveyed at each reef was not constant. Consequently, linear mixed effects models were chosen to examine the relationships between net carbonate production ( G ) and potential controls including the percentage cover of hard corals and macroalgae [33] , [34] ( Supplementary Tables S2 and S3 ). All modelling was performed in SPSS 19. Initially a saturated model was chosen, such that all sensible fixed and random effects of interest were included. The data were nested within reef and country and restricted maximum likelihood estimation was used to run the model. Thereafter, Akaike Information Criterion was used to select a suitable covariance structure and subsequently the best combination of random effects. This model was assessed graphically by examining a histogram of the standardized residuals to check for normality and by plotting the residuals versus the predicted values. Heterogeneity of variance was clear at this stage and the dependent variable (net carbonate production) was transformed: log (y+3). The model was run again with the transformed data as the dependent variable and the assumptions of normality and homogeneity of variance were confirmed. The fixed effects were then assessed by examining the significance of regression parameters [33] , [34] (see also Supplementary Methods ). Comparing contemporary and Holocene reef accretion rates To compare contemporary and Holocene reef accretion rates, rates of net carbonate production were converted to potential accretion rates (mm year −1 ) using established approaches based on carbonate density and framework porosity [15] , [21] , [22] . To account for the incorporation of bioerosion-derived sediment back into the reef structure, and thus as an addition to the reef accretion rate metric, we used a proportional sediment incorporation rate for the Caribbean of 50% based on data in ref. 21 . In this calculation we assumed that all urchin and endolithic sponge-derived erosional products, and 50% of parrotfish-derived erosional products (as a mobile taxa that defecates both on areas of reef framework and into sand channels) were available for potential incorporation. Comparisons with Holocene reef accretion rates in the Caribbean were based on the depth and habitat-stratified reef core data sets published in Hubbard [23] . How to cite this article: Perry, C. T. et al . Caribbean-wide decline in carbonate production threatens coral reef growth. Nat. Commun. 4:1402 doi: 10.1038/ncomms2409 (2013).